The amniote paratympanic organ develops from a previously undiscovered sensory placode The paratympanic organ, a mechanosensory hair cell-containing pouch in the amniote middle ear, was first described 100 years ago, yet its origins remain unresolved. Homology with the anamniote spiracular organ is supported by association with homologous skeletal elements and similar central targets of afferent neurons, suggesting it might be a remnant of the water-dependent lateral line system, otherwise lost during the amniote transition to terrestrial life. However, this is incompatible with studies suggesting that it arises from the first epibranchial (geniculate) placode. Here we show that a previously undiscovered Sox2-positive placode, immediately dorsal to the geniculate placode, forms the paratympanic organ and its afferent neurons, which are molecularly and morphologically distinct from geniculate neurons. These data remove the only obstacle to accepting the homology of the paratympanic organ and spiracular organ. We hypothesize that the paratympanic organ/spiracular organ represents an ancient head ectoderm module, developmentally and evolutionarily independent of both lateral line and epibranchial placodes. Vertebrate mechanosensory hair cells transduce various stimuli via deflection of the stereociliary bundle on their apical surfaces. Inner ear hair cells are stimulated by sounds and linear/angular acceleration; lateral line hair cells respond to local water movement. Inner ear and lateral line hair cells, and their afferent neurons, develop, respectively, from otic and lateral line placodes (paired, thickened patches of neurogenic head ectoderm) [1] , [2] , [3] . The water flow-sensing lateral line system was lost during amniote evolution. However, in many amniote species (most birds, alligators, Sphenodon and possibly some mammals; Fig. 1a ), mechanosensory hair cells are also found in the paratympanic organ (PTO): a small epithelial pouch embedded in connective tissue in the wall of the middle ear cavity [4] . In birds, PTO hair cells may be stimulated by mechanical distortion of the organ as a whole via elastic ligaments connected to the tympanic membrane and columella [5] : the PTO lumen is filled with a mucous substance that could act as a cupula, deflecting the stereocilia of the hair cells in response to deformation of the sense organ [6] . This has led to the hypothesis that the PTO responds to changes in air pressure, perhaps functioning as a barometer or altimeter [4] . 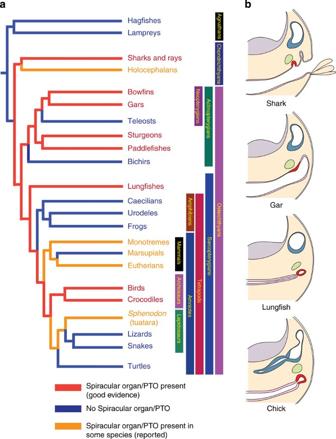Figure 1: A spiracular organ or PTO is found in many vertebrate groups. (a) Vertebrate phylogeny highlighting the presence of a spiracular organ or PTO, constructed using data from refs4,44,45. (NB Within the sarcopterygians, it is unknown whether or not coelacanths have a spiracular organ46, so they are not represented in the tree.) (b) Cartoons demonstrating similarities in the development of the spiracular organ and PTO (in association with the first pharyngeal pouch) in different species, drawn from our data plus refs36,47. Dark blue, inner ear epithelium; green, geniculate ganglion; red, spiracular organ/PTO; pink, pharyngeal endoderm; purple, neural tube. Figure 1: A spiracular organ or PTO is found in many vertebrate groups. ( a ) Vertebrate phylogeny highlighting the presence of a spiracular organ or PTO, constructed using data from refs 4 , 44 , 45 . (NB Within the sarcopterygians, it is unknown whether or not coelacanths have a spiracular organ [46] , so they are not represented in the tree.) ( b ) Cartoons demonstrating similarities in the development of the spiracular organ and PTO (in association with the first pharyngeal pouch) in different species, drawn from our data plus refs 36 , 47 . Dark blue, inner ear epithelium; green, geniculate ganglion; red, spiracular organ/PTO; pink, pharyngeal endoderm; purple, neural tube. Full size image It is unusual for hair cells to be activated by deformation of the sense organ itself, but the spiracular organ of cartilaginous fishes, non-teleost ray-finned fishes and lobe-finned fishes, which is embedded in connective tissue in the wall of the spiracle (that is, first pharyngeal slit), may operate in a similar manner. In sharks and skates, movement of the hyomandibula–cranial joint distorts the spiracular organ, triggering depolarization of spiracular organ hair cells (again perhaps via movement of a cupula), suggesting that it acts as a proprioceptor for jaw movement during feeding or intense respiration [7] , [8] , [9] . An evolutionary relationship between the PTO and spiracular organ is strongly supported: both are sense organs of the first pharyngeal cleft/pouch ( Fig. 1b ; the middle ear evolved from the spiracle), associated with homologous skeletal elements (the hyomandibula evolved into the columella/stapes of the tympanic middle ear [10] ). The spiracular organ is considered a specialized lateral line organ, and indeed spiracular organ afferents have been reported to project centrally to the mechanoreceptive lateral line nucleus and the vestibulocerebellum [7] , [8] , [9] . The amniote hindbrain lacks lateral nerve nuclei, but nerve-tracing experiments showed that PTO afferents project to vestibular nuclei and the cerebellum [11] , leading to the proposal that the PTO may represent a 'lateral line remnant' in amniotes [11] . However, fate-mapping experiments and clonal analysis in the chick [12] , [13] suggested that the PTO and its afferent neurons arise from the geniculate placode, the most rostral of the otherwise exclusively neurogenic epibranchial series of placodes lying dorsocaudal to each pharyngeal cleft (first, geniculate; second, petrosal; third and more caudal, nodose). Nerve-tracing experiments further showed that PTO afferent neurons reside in the geniculate ganglion and its so-called 'paratympanic extension' (a small nearby ganglion) [11] . If the PTO and spiracular organ are homologous, they should share a developmental lineage. The failure to reconcile the strong arguments for PTO/spiracular organ homology with the proposal that the PTO is geniculate placode-derived led us to examine the molecular development of the PTO for the first time since its discovery a century ago [14] . We show that the chicken PTO and its distinct afferent neurons are generated from a Sox2-positive placode immediately dorsal to and developmentally independent of the geniculate placode. We conclude that the PTO and spiracular organ are indeed homologous, and suggest that these sense organs and the placode from which they arise may be developmentally and evolutionarily independent of both epibranchial and lateral line placodes. Sense organs of the first pharyngeal cleft Histological analysis of spiracular organ development in the lesser-spotted dogfish (catshark), Scyliorhinus canicula , highlighted the developmental similarities with the PTO in chicken embryos. The chicken PTO is embedded in connective tissue within the wall of the middle ear cavity (derived from the first pharyngeal cleft), in close proximity to the tympanic membrane ( Fig. 2a,b ). In the shark, the maturing spiracular organ is positioned in the dorsal wall of the first gill slit (spiracle) ( Fig. 2c,d ). Both sense organs possess mechanosensory hair cells, organized unilaterally into columnar epithelia ( Fig. 2b,c ). During chicken embryogenesis, the PTO can be identified as an ectodermal condensation at the lateral tip of the first pharyngeal pouch, immediately ventral to the jugular vein ( Fig. 2e ). In S. canicula , the forming spiracular organ can similarly be observed as an epithelial pouch associated with the first gill pouch endoderm, ventral to the jugular vein ( Fig. 2f ). The ectodermal origin of the PTO [12] was confirmed using isotopic quail-chick grafts of prospective peri-geniculate placode region ectoderm (that is, ectoderm associated with the first pharyngeal cleft). As expected [12] this labelled the PTO, including the hair cells within it (detected by immunostaining for the hair cell-specific structural marker myosin VIIa), as well as neurons in both the geniculate ganglion and its 'paratympanic extension' ( Fig. 2g–i ). 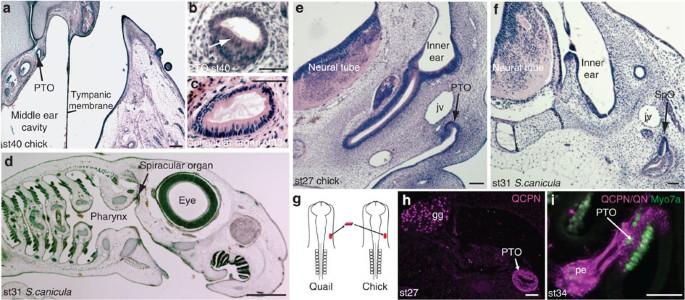Figure 2: Sense organs of the first pharyngeal pouch. (a) Transverse haematoxylin and eosin (H&E)-stained section of stage 40 (E14) chicken head highlighting position of PTO and tympanic membrane. (b) Magnified view of PTO at stage 40 (E14). Mechanosensory hair cells (arrow) line the medial wall. (c) Transverse H&E-stained section of shark spiracular organ at stage 33 (16–22 weeks). (d) Parasagittal section of shark head at stage 31 (60–80 days), highlighting the position of the spiracular organ in the first pharyngeal cleft. (e) Transverse section of stage 27 (E5) chicken embryo; the developing PTO is indicated at the tip of the first pharyngeal pouch. (f) Transverse section of stage 31 shark embryo (60–80 days). The forming spiracular organ is associated with the first pharyngeal cleft. (g) Schematic representation of isotopic quail/chick grafting procedure; excised quail ectoderm is transplanted to an equivalent position in chick hosts. (h) Transverse section of chimeric embryo following isotopic grafting. Quail cells are labelled with QCPN antibody (magenta) and contribute extensively to the PTO and geniculate ganglion (gg). (i) Magnified view of chimeric PTO at stage 34 (E8) demonstrating quail-derived hair cells and neurons of the 'paratympanic extension of the geniculate ganglion' (pe). Scale bars, 100 μm (a); 50 μm (b,c,e,f,h,i); 500 μm (d). Myo7a, myosin VIIa (hair cell-specific marker); QCPN, quail-specific antibody (recognizes peri-nuclear antigen); QN, quail neurite-specific antibody. Figure 2: Sense organs of the first pharyngeal pouch. ( a ) Transverse haematoxylin and eosin (H&E)-stained section of stage 40 (E14) chicken head highlighting position of PTO and tympanic membrane. ( b ) Magnified view of PTO at stage 40 (E14). Mechanosensory hair cells (arrow) line the medial wall. ( c ) Transverse H&E-stained section of shark spiracular organ at stage 33 (16–22 weeks). ( d ) Parasagittal section of shark head at stage 31 (60–80 days), highlighting the position of the spiracular organ in the first pharyngeal cleft. ( e ) Transverse section of stage 27 (E5) chicken embryo; the developing PTO is indicated at the tip of the first pharyngeal pouch. ( f ) Transverse section of stage 31 shark embryo (60–80 days). The forming spiracular organ is associated with the first pharyngeal cleft. ( g ) Schematic representation of isotopic quail/chick grafting procedure; excised quail ectoderm is transplanted to an equivalent position in chick hosts. ( h ) Transverse section of chimeric embryo following isotopic grafting. Quail cells are labelled with QCPN antibody (magenta) and contribute extensively to the PTO and geniculate ganglion (gg). ( i ) Magnified view of chimeric PTO at stage 34 (E8) demonstrating quail-derived hair cells and neurons of the 'paratympanic extension of the geniculate ganglion' (pe). Scale bars, 100 μm ( a ); 50 μm ( b , c , e , f , h , i ); 500 μm ( d ). Myo7a, myosin VIIa (hair cell-specific marker); QCPN, quail-specific antibody (recognizes peri-nuclear antigen); QN, quail neurite-specific antibody. Full size image The PTO anlage is molecularly distinct The transcription factor Sox2 is essential for mechanosensory hair-cell formation and is one of the earliest indicators of prosensory bias in the inner ear [15] . At Hamburger–Hamilton stage 18 (65–69 h of development [16] ), we discovered a patch of Sox2 -positive ectoderm ( Fig. 3a,b ) dorsal to the geniculate placode, which we identified by Pax2 , Sox3 and Delta1 expression [1] ( Fig. 3c–e ). At earlier stages, Pax2 and Sox3 are expressed throughout the 'posterior placodal area', a common ectodermal domain from which the otic and epibranchial placodes develop [3] , [17] ; their expression subsequently resolves to the otic and epibranchial placodes [17] . In Xenopus , the posterior placodal area, which expresses Sox2 as well as Sox3 , gives rise to lateral line, otic and epibranchial placodes; Sox2 expression is gradually lost from the epibranchial placodes, but both Sox2 and Sox3 persist strongly in the otic and lateral line placodes [3] , [18] . In the chick at stage 14 (50–53 h), when neuroblasts are just starting to delaminate from the geniculate placode [12] , double immunostaining on tissue sections at the level of the first pharyngeal cleft revealed Sox2 expression in some cells in the dorsalmost region of Sox3-positive ectoderm (arrow, Fig. 3f ), and, much more weakly, in a subset of more ventral Sox3-positive cells. At stage 18 (65–69 h), when neuroblast emigration from the geniculate placode is at its peak [12] , and also a few hours later at stage 20 (70–72 h), strong Sox2 expression is seen in a discrete domain of thickened ectoderm immediately dorsal to the Sox3-positive geniculate placode (arrow, Fig. 3g,h ), a subset of whose cells still weakly co-express Sox2. Most of the strongly Sox2-positive, dorsally located cells appear not to express Sox3 ( Fig. 3g,h ). (Sox2-positive cells in the mesenchyme are neural crest-derived neuroglial progenitors associated with the developing geniculate ganglion [19] .) At stages 22 (E3.5) and 24 (E4), a strongly Sox2-positive patch of thickened ectoderm is located immediately dorsal to the strongly Sox3-positive, Sox2-negative remnant of the geniculate placode (arrow, Fig. 3i,j ). Weak Sox3 expression is also seen in many of the Sox2-positive dorsal cells at these stages, perhaps correlating with the onset of neurogenesis in this dorsal patch of Sox2-positive ectoderm from stages 22/23 (E3.5–4) (see below). Double immunostaining for Sox2 and Pax2 at stage 24 (E4) reveals a similar picture, that is, a strongly Sox2-positive patch of thickened ectoderm immediately dorsal to the Pax2-positive, Sox2-negative geniculate placode remnant ( Fig. 3k ). 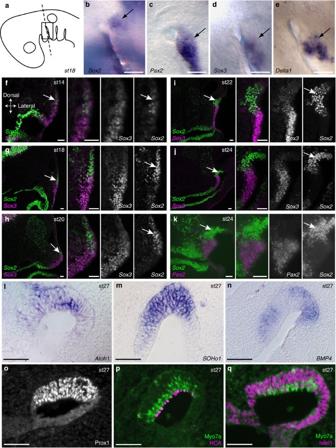Figure 3: A distinct PTO placode. (a) Schematic indicating the approximate locations of whole mount images in panelsb–e(box), and approximate plane of section for images in panelsf–q(dotted line). (b) Whole mountSox2 in situhybridization at stage 18 (65–69 h) reveals a patch ofSox2-positive ectoderm (putative PTO placode, arrow) at the dorsocaudal edge of the first pharyngeal cleft. (c–e) Whole mountin situhybridization for the epibranchial placode markersPax2,Sox3andDelta1at stage 18 (65–69 h). (f–j) Transverse sections at the level shown in panela, immunostained for Sox2 (green) and Sox3 (magenta), at stages 14 (50–53 h), 18 (65–69 h), 20 (70–72 h), 22 (E3.5) and 24 (E4). (k) Transverse section at the level shown in panela, immunostained for Sox2 and Pax2, at stage 24 (E4). (l–q)In situhybridization or immunostaining on sections of the PTO at stage 27 (E5) reveals expression of typical hair cell/sensory patch-associated markers (Atoh1,SOHo1,BMP4and Prox1) and the hair cell-specific structural markers myosin VIIA (Myo7a) and Ptprq/HCA. Scale bars, 50 μm. Figure 3: A distinct PTO placode. ( a ) Schematic indicating the approximate locations of whole mount images in panels b – e (box), and approximate plane of section for images in panels f – q (dotted line). ( b ) Whole mount Sox2 in situ hybridization at stage 18 (65–69 h) reveals a patch of Sox2 -positive ectoderm (putative PTO placode, arrow) at the dorsocaudal edge of the first pharyngeal cleft. ( c – e ) Whole mount in situ hybridization for the epibranchial placode markers Pax2 , Sox3 and Delta1 at stage 18 (65–69 h). ( f – j ) Transverse sections at the level shown in panel a , immunostained for Sox2 (green) and Sox3 (magenta), at stages 14 (50–53 h), 18 (65–69 h), 20 (70–72 h), 22 (E3.5) and 24 (E4). ( k ) Transverse section at the level shown in panel a , immunostained for Sox2 and Pax2, at stage 24 (E4). ( l – q ) In situ hybridization or immunostaining on sections of the PTO at stage 27 (E5) reveals expression of typical hair cell/sensory patch-associated markers ( Atoh1 , SOHo1 , BMP4 and Prox1) and the hair cell-specific structural markers myosin VIIA (Myo7a) and Ptprq/HCA. Scale bars, 50 μm. Full size image During embryonic day 4, the Sox2-positive PTO placodal ectoderm, together with the Pax2-positive/Sox3-positive remnant of the geniculate placode, is internalized (for example, Fig. 3j ) such that by stage 27 (E5), the Sox2-positive PTO ectoderm resides at the tip of the pharyngeal pouch ( Supplementary Fig. S1 ). (The internalization and fusion of epibranchial placodes with pharyngeal pouch endoderm, and subsequent loss of connection with the ectoderm, has long been known, for example, ref. 20 .) Also from stage 27 (E5), we detected expression within the Sox2-positive PTO ectoderm of Atoh1 , encoding a transcription factor essential for hair cell development [21] ( Fig. 3l ) plus other genes characteristic of inner ear sensory organ formation, such as SOHo1 , BMP4 and Prox1 ( Fig. 3m–o ), and hair cell-specific structural markers including the non-muscle myosin VIIA, and Ptprq (hair cell antigen, HCA) ( Fig. 3p,q ). From stage 29 (E6), the PTO begins to separate from the pharyngeal pouch epithelium to form a vesicle. At this stage, we saw strong immunoreactivity for activated caspase 3 (arrow, Supplementary Fig. S1d,e ) and apoptotic bodies ( Supplementary Fig. S1f ) in a localized area of pharyngeal epithelium medial to the developing PTO. This localized apoptosis is presumably important for the separation of the PTO from the pharyngeal pouch epithelium. We conclude that strong Sox2 expression defines a discrete region of thickened ectoderm, lying immediately dorsal to the geniculate placode, from which the PTO is generated. Hence, the PTO placode is molecularly and spatially distinct from the adjacent geniculate placode. Although there is no clear morphological distinction between the PTO and geniculate placodes, we note that in at least some anamniotes the border between epibranchial placodes and adjacent lateral line placodes cannot always be distinguished morphologically (for example, refs 22 , 23 , 24 ). The PTO generates its own distinct afferent neurons The differences described above between geniculate placode and PTO development were reinforced by our discovery that the PTO generates its own afferent neurons. The peak delamination of geniculate placode-derived neurons occurs around stages 17–18 (52–69 h [12] ). We observed that the Sox2-positive PTO placode contributes a previously unreported population of sensory neurons to the geniculate ganglion. These PTO neurons specifically express the vestibuloacoustic neuron marker Brn3a and begin to delaminate from the Sox2-positive PTO placode from stages 22/23 (E3.5-4); no Brn3a-positive cells were detectable at earlier stages in this region (for example, Fig. 4a–e ). We note that Sox3, which is necessary for neurogenesis in the chick otic vesicle and epibranchial placodes [25] , [26] , seems to be upregulated in a subset of PTO placode cells from stage 22 (E3.5) onwards ( Fig. 3i,j ), perhaps correlating with the onset of neurogenesis in the PTO placode. At stage 24 (E4), Brn3a expression is confined to delaminated PTO neuroblasts, many of which can be seen immediately adjacent to a region of the PTO epithelium apparently devoid of laminin immunostaining ( Fig. 4f–j ). At stage 27 (E5), many Brn3a-positive cells are also present within the PTO epithelium, and Brn3a-positive neurons can be seen delaminating though breaches in the basement membrane ( Fig. 4k–o ). Delaminated PTO neurons migrate towards the geniculate ganglion and initially populate its proximal region ( Fig. 4k , arrow), but do not express the epibranchial neuron marker Phox2b ( Fig. 5a–c ). By stage 31 (E7), Brn3a-positive neurons are still detectable in the geniculate ganglion ( Fig. 5d,e ) and in a small, separate ganglion previously termed the 'paratympanic extension of the geniculate ganglion' ( Fig. 5e ). These data are consistent both with previous nerve-tracing experiments [11] and also with retroviral lineage-labelling experiments suggesting a clonal relationship (hence, common origin) between PTO hair cells and some neurons in the geniculate ganglion [13] . By stage 35 (E9), neurons in the PTO ganglion are not only molecularly distinct but also significantly smaller than geniculate neurons (mean diameter 12.6±1.5 μm versus 18.1±1.8 μm, respectively, P <0.001, Student's t -test; Fig. 5f–i ). 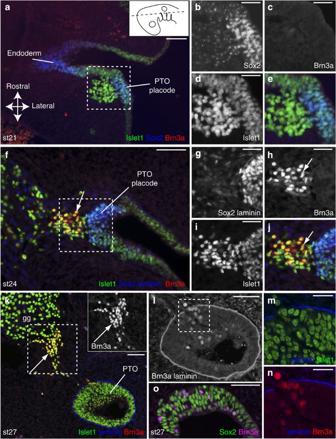Figure 4: The PTO placode gives rise to Brn3a-positive neurons. (a) Coronal section of PTO placode at stage 21 (E3.5), immunostained for the PTO placode marker Sox2 (blue), the neuronal marker Islet1 (green) and Brn3a (red). Dotted line on schematic insert indicates plane of section; axes indicated with arrows. (b–e) Magnified view of the boxed area in panelashowing single channel and merged images. No Brn3a-positive cells are present at this stage. (f) Coronal section of PTO placode at stage 24 (E4), immunostained for Sox2 (blue), laminin (blue), Islet1 (green) and Brn3a (red). Brn3a-positive neurons (arrow) are closely associated with the Sox2-positive PTO placode. (g–j) Single channel and merged images of magnified view of boxed region in panelf, highlighting Brn3a-positive neurons (arrow) adjacent to a large breach in the basement membrane of the Sox2-positive PTO placode. (k) Coronal section of PTO at stage 27 (E5), immunostained for laminin (blue), Islet1 (green) and Brn3a (red). A discrete cluster of Brn3a-positive neurons (arrow) seem to be merging with the edge of the geniculate ganglion closest to the PTO. (l) Magnified view of PTO from panelk, showing both Brn3a and laminin in greyscale for clarity. Brn3a-positive cells can be seen delaminating from the PTO through gaps in the basement membrane. (m,n) Magnified view of boxed region from panell, highlighting the delamination of Brn3a-positive cells. (o) Coronal section of PTO at stage 27 (E5), immunostained for Sox2 (green) and Brn3a (magenta), confirming the persistence of Sox2 protein in the PTO epithelium. Brn3a-positive cells are scattered throughout the epithelium. Scale bars, 50 μm (a,f,k,l,o); 25 μm (b–e,g–j,m,n). Figure 4: The PTO placode gives rise to Brn3a-positive neurons. ( a ) Coronal section of PTO placode at stage 21 (E3.5), immunostained for the PTO placode marker Sox2 (blue), the neuronal marker Islet1 (green) and Brn3a (red). Dotted line on schematic insert indicates plane of section; axes indicated with arrows. ( b – e ) Magnified view of the boxed area in panel a showing single channel and merged images. No Brn3a-positive cells are present at this stage. ( f ) Coronal section of PTO placode at stage 24 (E4), immunostained for Sox2 (blue), laminin (blue), Islet1 (green) and Brn3a (red). Brn3a-positive neurons (arrow) are closely associated with the Sox2-positive PTO placode. ( g – j ) Single channel and merged images of magnified view of boxed region in panel f , highlighting Brn3a-positive neurons (arrow) adjacent to a large breach in the basement membrane of the Sox2-positive PTO placode. ( k ) Coronal section of PTO at stage 27 (E5), immunostained for laminin (blue), Islet1 (green) and Brn3a (red). A discrete cluster of Brn3a-positive neurons (arrow) seem to be merging with the edge of the geniculate ganglion closest to the PTO. ( l ) Magnified view of PTO from panel k , showing both Brn3a and laminin in greyscale for clarity. Brn3a-positive cells can be seen delaminating from the PTO through gaps in the basement membrane. ( m , n ) Magnified view of boxed region from panel l , highlighting the delamination of Brn3a-positive cells. ( o ) Coronal section of PTO at stage 27 (E5), immunostained for Sox2 (green) and Brn3a (magenta), confirming the persistence of Sox2 protein in the PTO epithelium. Brn3a-positive cells are scattered throughout the epithelium. Scale bars, 50 μm ( a , f , k , l , o ); 25 μm ( b – e , g – j , m , n ). 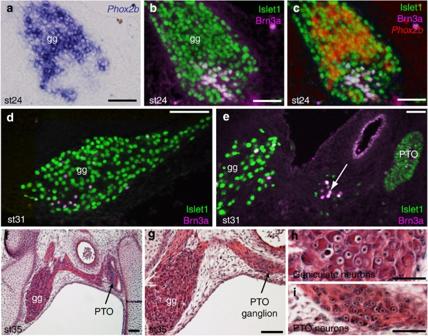Figure 5: PTO neurons populate the geniculate ganglion and also form a separate PTO ganglion. (a) Transverse section of geniculate ganglion at stage 24 (E4), followingPhox2b in situhybridization to label epibranchial neurons. (b) Same section immunostained for Brn3a (magenta) and Islet1 (green), showing a cluster of Brn3a-positive neurons towards the edge of the geniculate ganglion in a region that (by comparison with panela) seemsPhox2b-negative. (c) Pseudo-coloured overlay of panelsaandbhighlighting the apparent segregation of Brn3a-positive andPhox2b-positive neurons. (d) Transverse section of geniculate ganglion at stage 31 (E7) immunostained for Brn3a (magenta) and Islet1 (green). Brn3a-positive neurons are still present within the geniculate ganglion. (e) A different transverse section at stage 31 (E7), immunostained for Brn3a (magenta) and Islet1 (green), showing that Brn3a-positive neurons are also detected in a small cluster between the PTO and geniculate ganglion (arrow). This PTO ganglion was previously described as the 'paratympanic extension of the geniculate ganglion'. (f) At stage 35 (E9), H&E staining shows the axonal tracts connecting the geniculate ganglion and PTO. (g) The PTO ganglion resides within this axonal tract. (h,i) Magnified views of neuronal cell bodies within the geniculate ganglion and PTO ganglion, respectively, highlighting the smaller diameter of the PTO neurons. Scale bars, 100 μm (a–g); 50 μm (h,i). gg, geniculate ganglion. Full size image Figure 5: PTO neurons populate the geniculate ganglion and also form a separate PTO ganglion. ( a ) Transverse section of geniculate ganglion at stage 24 (E4), following Phox2b in situ hybridization to label epibranchial neurons. ( b ) Same section immunostained for Brn3a (magenta) and Islet1 (green), showing a cluster of Brn3a-positive neurons towards the edge of the geniculate ganglion in a region that (by comparison with panel a ) seems Phox2b -negative. ( c ) Pseudo-coloured overlay of panels a and b highlighting the apparent segregation of Brn3a-positive and Phox2b -positive neurons. ( d ) Transverse section of geniculate ganglion at stage 31 (E7) immunostained for Brn3a (magenta) and Islet1 (green). Brn3a-positive neurons are still present within the geniculate ganglion. ( e ) A different transverse section at stage 31 (E7), immunostained for Brn3a (magenta) and Islet1 (green), showing that Brn3a-positive neurons are also detected in a small cluster between the PTO and geniculate ganglion (arrow). This PTO ganglion was previously described as the 'paratympanic extension of the geniculate ganglion'. ( f ) At stage 35 (E9), H&E staining shows the axonal tracts connecting the geniculate ganglion and PTO. ( g ) The PTO ganglion resides within this axonal tract. ( h , i ) Magnified views of neuronal cell bodies within the geniculate ganglion and PTO ganglion, respectively, highlighting the smaller diameter of the PTO neurons. Scale bars, 100 μm ( a – g ); 50 μm ( h , i ). gg, geniculate ganglion. Full size image We also performed a series of retrograde and anterograde dye-tracing experiments to determine the projection patterns of PTO afferent neurons ( Fig. 6 ). Overall, our results were consistent with a previous report [11] that PTO afferents project centrally as a distinct bundle within the facial nerve, and terminate overlappingly with vestibular fibres in vestibular nuclei ( Fig. 6 ). Retrograde tracing from the hindbrain at stage 28 (E5.5) showed the projection of PTO afferents as a bundle within the facial nerve ( Fig. 6a ) and revealed a unique PTO nerve [27] lying between the greater petrosal nerve and chorda tympani ( Fig. 6b,c ; this may be the postspiracular branch of the facial nerve described in ref. 28 ). At stages 28–30 (E5.5–6.5), labelling from different combinations of the various nerves plus the inner ear showed overlapping projection of PTO afferents with inner ear afferents ( Fig. 6d–j ). In contrast, gustatory, general viscerosensory and somatosensory afferents from the geniculate ganglion enter the hindbrain in the facial nerve and terminate, respectively, in the solitary tract (gustatory, general viscerosensory) and descending trigeminal tract (somatosensory) ( Fig. 6d,j ). These data are summarized in schematic form in Fig. 6k,l . 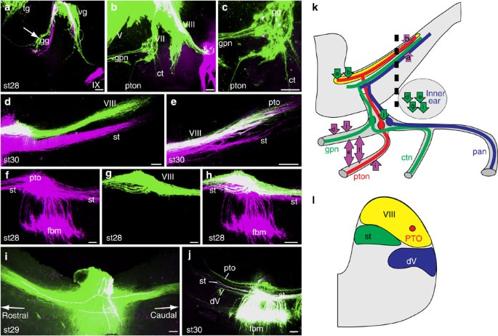Figure 6: Central projections of the PTO nerve overlap with inner ear afferents. Approximate dye-insertion sites indicated by corresponding arrows in panelk; magenta/green overlap shows as white. (a) Retrograde tracing at stage 28 (E5.5) from the cerebellum (rhombomere 1/2 boundary) (green) plus a caudal dye insertion in the descending tract (magenta) shows projection of presumed PTO afferents as a distinct bundle within the facial nerve (arrow). gg, geniculate ganglion (VII); tg, trigeminal ganglion (V); vg, vestibuloacoustic ganglion (VIII). (b,c) Stage 28 (E5.5) ganglia backfilled from a rostral (green) and caudal (magenta) dye insertion into the hindbrain. In the geniculate ganglion, the rostral dye insertion (green) labelled fibres in the greater petrosal nerve (gpn) and chorda tympani (ct), and a unique nerve lying between them, the PTO nerve (pton). [The caudal dye insertion (magenta) labelled many afferents from the inner ear (VIII) and glossopharyngeal nerve (IX) but filled only a few geniculate ganglion neurons.] (c) Higher-power view of geniculate ganglion region fromb. (d) At stage 30 (E6.5), labelling from the greater petrosal nerve alone (magenta) plus the inner ear (green) shows no overlap with inner ear afferents (VIII). st, solitary tract. (e–h) In contrast, labelling from the greater petrosal and PTO nerves (magenta), plus the inner ear (green), shows extensive overlap with inner ear afferents (VIII) at stage 30 (E6.5;e) and stage 28 (E5.5;f–h). fbm, facial branchiomotor neurons. (i) At stage 29 (E6), labelling from the PTO nerve (magenta) and inner ear (green) likewise shows projection of PTO afferents with inner ear afferents (VIII). (j) At stage 30 (E6.5), sequential labelling from the greater petrosal nerve (magenta) plus the geniculate ganglion (green) shows overlapping afferents in the solitary tract (st): the descending trigeminal tract (dV) and PTO afferents are only labelled with the geniculate ganglion dye insertion (green). (k) Schematic showing the peripheral and central distribution of geniculate ganglion afferents: gustatory/viscerosensory afferents (green) to the greater petrosal (gpn) and chorda tympani (ctn) nerves and solitary tract; somatosensory afferents (blue) to the posterior auricular nerve (pan) and the descending tract of the trigeminal; PTO afferents (red) to the inner ear projection (yellow, VIII). (l) Coronal section at the approximate position indicated by the dashed line in panelk. Scale bars, 100 μm. Figure 6: Central projections of the PTO nerve overlap with inner ear afferents. Approximate dye-insertion sites indicated by corresponding arrows in panel k ; magenta/green overlap shows as white. ( a ) Retrograde tracing at stage 28 (E5.5) from the cerebellum (rhombomere 1/2 boundary) (green) plus a caudal dye insertion in the descending tract (magenta) shows projection of presumed PTO afferents as a distinct bundle within the facial nerve (arrow). gg, geniculate ganglion (VII); tg, trigeminal ganglion (V); vg, vestibuloacoustic ganglion (VIII). ( b , c ) Stage 28 (E5.5) ganglia backfilled from a rostral (green) and caudal (magenta) dye insertion into the hindbrain. In the geniculate ganglion, the rostral dye insertion (green) labelled fibres in the greater petrosal nerve (gpn) and chorda tympani (ct), and a unique nerve lying between them, the PTO nerve (pton). [The caudal dye insertion (magenta) labelled many afferents from the inner ear (VIII) and glossopharyngeal nerve (IX) but filled only a few geniculate ganglion neurons.] ( c ) Higher-power view of geniculate ganglion region from b . ( d ) At stage 30 (E6.5), labelling from the greater petrosal nerve alone (magenta) plus the inner ear (green) shows no overlap with inner ear afferents (VIII). st, solitary tract. ( e – h ) In contrast, labelling from the greater petrosal and PTO nerves (magenta), plus the inner ear (green), shows extensive overlap with inner ear afferents (VIII) at stage 30 (E6.5; e ) and stage 28 (E5.5; f – h ). fbm, facial branchiomotor neurons. ( i ) At stage 29 (E6), labelling from the PTO nerve (magenta) and inner ear (green) likewise shows projection of PTO afferents with inner ear afferents (VIII). ( j ) At stage 30 (E6.5), sequential labelling from the greater petrosal nerve (magenta) plus the geniculate ganglion (green) shows overlapping afferents in the solitary tract (st): the descending trigeminal tract (dV) and PTO afferents are only labelled with the geniculate ganglion dye insertion (green). ( k ) Schematic showing the peripheral and central distribution of geniculate ganglion afferents: gustatory/viscerosensory afferents (green) to the greater petrosal (gpn) and chorda tympani (ctn) nerves and solitary tract; somatosensory afferents (blue) to the posterior auricular nerve (pan) and the descending tract of the trigeminal; PTO afferents (red) to the inner ear projection (yellow, VIII). ( l ) Coronal section at the approximate position indicated by the dashed line in panel k . Scale bars, 100 μm. Full size image Overall, our data suggest that the avian PTO and its afferent neurons are generated from a molecularly distinct PTO placode located immediately dorsal to the geniculate placode, and not from the geniculate placode as previously thought. Furthermore, PTO afferent neurons are molecularly and morphologically distinct from geniculate placode-derived neurons, and show distinctive projection patterns. Dissociable competence to form PTO versus geniculate placode We used quail-chick chimeras to assay the competence of different ectodermal tissues to form geniculate neurons versus the PTO ( Fig. 7a ). Control isotopic grafts of quail peri-geniculate region ectoderm contributed as expected [11] , [12] , [13] to geniculate neurons, the PTO itself and Brn3a-positive PTO neurons ( Fig. 7b–d ). Heterotopic transplants into the peri-geniculate region revealed that competence to form the PTO is experimentally dissociable from competence to form geniculate neurons. Otic placode ectoderm from 5–10 somite stage (ss) quail donors was competent to form both geniculate neurons and hair cells in the PTO ( n =2/4). Prospective nodose (third epibranchial) placode ectoderm (located lateral to the first 2 somites [12] ) from 1–12ss donors always contributed neurons to the geniculate ganglion, but in only 1/9 cases (from a 5ss donor) contributed to the PTO, including hair cells. (We used isotopic grafts to confirm that this ectoderm normally contributes neurons to the nodose ganglion and does not normally contribute to the geniculate ganglion or PTO; n =5.) Prospective trigeminal placode ectoderm (taken lateral to rhombomeres 1, 2 at the 5–10ss [12] , [29] ) formed geniculate neurons but did not contribute cells to the PTO ( n =4). Similar results were obtained with trunk ectoderm (taken lateral to the most caudal 2–3 somites of 8–11ss donor embryos), which always formed neurons in the geniculate ganglion (as expected, given that trunk ectoderm is competent to form nodose neurons [30] ) but failed to contribute cells to the PTO ( n =10; Fig. 7e ). This difference in competence also held true for the formation of Brn3a-positive PTO neurons ( Fig. 7f,g ): trunk ectoderm efficiently generated geniculate neurons, but only 1/202 (0.5%) quail neurons in the geniculate ganglion across four embryos was scored as Brn3a-positive. In contrast, control grafts of peri-geniculate region ectoderm readily generated Brn3a-positive neurons in the geniculate ganglion (154/245 cells: 63%, across two embryos). This suggests not only that competence to form the PTO is much more restricted spatially than competence to form the geniculate placode, but that Brn3a-positive cells in the geniculate and PTO ganglia are exclusively derived from the PTO placode. These data also rule out a 'temporal segregation' model in which the geniculate placode first forms geniculate neurons, and later forms PTO neurons and the PTO, as this model would predict that ectoderm competent to form geniculate neurons should also be competent to form PTO neurons and the PTO. Instead, our results suggest that the induction of the geniculate placode and the PTO is not tightly coupled, which is also consistent with the evolutionary loss specifically of the PTO (without any effect on the geniculate ganglion) in multiple lineages ( Fig. 1a ). 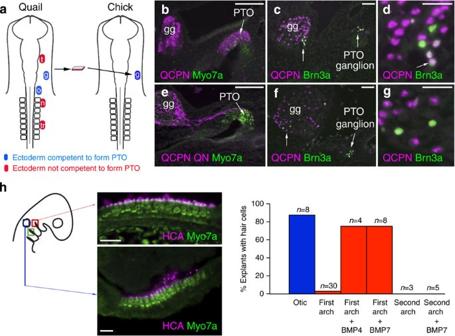Figure 7: Competence to form the PTO and PTO neurons is dissociable from competence to form geniculate neurons. (a) Schematic summarizing grafting of different regions of quail ectoderm into the peri-geniculate placode region of chicken hosts. Grafts from blue regions—prospective peri-geniculate (g) and otic (o) placodes—were competent to form both geniculate neurons and the PTO. Grafts from red regions—presumptive trigeminal placode (t), nodose placode (n) and trunk ectoderm (t)—were competent to form geniculate neurons but not the PTO. (b–d) Transverse sections through the PTO region of chimeric embryos after control isotopic grafts of quail peri-geniculate region ectoderm, immunostained for the quail perinuclear antigen (QCPN), the hair cell marker myosin VIIA (Myo7) and Brn3a, showing that peri-geniculate ectoderm contributes as expected to geniculate neurons, the PTO and Brn3a-positive PTO neurons. (e) In contrast, trunk ectoderm is competent to form geniculate neurons, but not the PTO. Similar results were obtained after grafting prospective trigeminal or nodose placode ectoderm. (f,g) Trunk ectoderm grafts also fail to form Brn3a-positive PTO neurons in either the geniculate or PTO ganglia. (h)In vitroculture of tissue from the otocyst generates hair cells after 5–7 days in floating culture (blue box in embryo schematic; lower panel showing cryosection immunostained for hair cell markers; blue bar in bar chart). Tissue from the peri-geniculate placode region (first pharyngeal cleft) generates hair cells in floating culture only in the presence of BMPs (red box in embryo schematic; upper panel showing cryosection immunostained for hair cell markers; red bars in bar chart). Tissue from the peri-petrosal placode region (second pharyngeal cleft) does not generate hair cells even in the presence of BMPs (green box in embryo schematic; see bar chart for quantification), confirming the restriction of PTO-forming competence to the peri-geniculate region. Scale bars, 100 μm (b,c,e,f); 50 μm (d,g); 20 μm (h). Myo7a, myosin VIIa. Figure 7: Competence to form the PTO and PTO neurons is dissociable from competence to form geniculate neurons. ( a ) Schematic summarizing grafting of different regions of quail ectoderm into the peri-geniculate placode region of chicken hosts. Grafts from blue regions—prospective peri-geniculate (g) and otic (o) placodes—were competent to form both geniculate neurons and the PTO. Grafts from red regions—presumptive trigeminal placode (t), nodose placode (n) and trunk ectoderm (t)—were competent to form geniculate neurons but not the PTO. ( b – d ) Transverse sections through the PTO region of chimeric embryos after control isotopic grafts of quail peri-geniculate region ectoderm, immunostained for the quail perinuclear antigen (QCPN), the hair cell marker myosin VIIA (Myo7) and Brn3a, showing that peri-geniculate ectoderm contributes as expected to geniculate neurons, the PTO and Brn3a-positive PTO neurons. ( e ) In contrast, trunk ectoderm is competent to form geniculate neurons, but not the PTO. Similar results were obtained after grafting prospective trigeminal or nodose placode ectoderm. ( f , g ) Trunk ectoderm grafts also fail to form Brn3a-positive PTO neurons in either the geniculate or PTO ganglia. ( h ) In vitro culture of tissue from the otocyst generates hair cells after 5–7 days in floating culture (blue box in embryo schematic; lower panel showing cryosection immunostained for hair cell markers; blue bar in bar chart). Tissue from the peri-geniculate placode region (first pharyngeal cleft) generates hair cells in floating culture only in the presence of BMPs (red box in embryo schematic; upper panel showing cryosection immunostained for hair cell markers; red bars in bar chart). Tissue from the peri-petrosal placode region (second pharyngeal cleft) does not generate hair cells even in the presence of BMPs (green box in embryo schematic; see bar chart for quantification), confirming the restriction of PTO-forming competence to the peri-geniculate region. Scale bars, 100 μm ( b , c , e , f ); 50 μm ( d , g ); 20 μm ( h ). Myo7a, myosin VIIa. Full size image The restriction of PTO-forming competence to the peri-geniculate region was further confirmed by showing that exogenous bone morphogenetic proteins (BMPs) promote hair cell differentiation from cultured first pharyngeal cleft tissue (which includes the geniculate placode and PTO placode) but not second pharyngeal cleft tissue, which includes the petrosal (second epibranchial) placode ( Fig. 7h ). We successfully cultured hair cells, identified both by morphology and double immunostaining for the hair cell-specific structural markers myosin VIIa and Ptprq/HCA, from stage 15–16 (24–28ss) chicken otocyst explants ( n =7/8). Under identical conditions, only 3% ( n =1/30) of stage 15–16 tissue explants from the first pharyngeal cleft region (comprising geniculate and PTO placode region ectoderm, mesoderm and endoderm) produced hair cells. However, a significant proportion of first pharyngeal cleft explant cultures produced hair cells when the defined culture medium was supplemented with either BMP4 (75%; n =3/4) or BMP7 (75%; n =6/8). In contrast, similar tissue explants from the second pharyngeal cleft region, that is, petrosal (second epibranchial) placode region ectoderm, plus underlying mesoderm and endoderm, failed to generate any hair cells, either when cultured alone ( n =0/3) or when supplemented with BMP7 ( n =0/5) ( Fig. 7h ). Hence, peri-geniculate region ectoderm (that is, PTO placode plus geniculate placode) is competent to generate hair cells when cultured with BMPs, whereas petrosal placode ectoderm is not. Our results indicate that the avian PTO and its afferent neurons are derived from a previously undiscovered placode that is molecularly and spatially distinct from and developmentally independent of the adjacent geniculate placode. This conclusion is retrospectively supported by peri-geniculate placode ectoderm ablation experiments performed almost 70 years ago by Yntema [27] : in most cases this led only to a reduction in size, rather than loss, of the geniculate ganglion, but had a significant effect on the PTO, which was either missing entirely, or had fewer or no hair cells. These results suggest that while the geniculate placode is relatively easily regenerated following ablation, the PTO placode is not. Our data also show that PTO afferent neurons are molecularly and morphologically distinct from geniculate placode-derived neurons; they form a unique peripheral nerve, project into the hindbrain as a distinct bundle within the facial nerve and differ in their central projection patterns. The demonstration that the PTO and its afferent neurons develop from a unique placode immediately dorsal to the geniculate placode, and not from the geniculate placode itself as previously thought [12] , [13] , removes the only obstacle to acceptance of the previously proposed homology of the PTO with the anamniote spiracular organ (based on position, morphology, association with homologous skeletal elements and similar central projection patterns of afferent neurons [5] , [9] , [11] , [31] ). Although the spiracular organ has been considered a specialized lateral line organ, its developmental origin remains unclear. Spiracular organ afferents reside in the otic lateral line ganglion and project via the otic lateral line nerve to lateral line nuclei [32] , suggesting that the spiracular organ is otic lateral line placode-derived. If the PTO is homologous with the spiracular organ, this would in turn suggest that the PTO derives from a remnant otic lateral line placode. However, our data demonstrate that molecularly distinct PTO neurons originate from a unique placode, but join the geniculate ganglion and project via the facial nerve to the vestibular nuclei. Therefore, a more complex development for the spiracular organ and its afferent neurons cannot be excluded. Indeed, reports from a shark [33] (cartilaginous fish) and two species of gars (non-teleost ray-finned fishes) [34] , [35] suggest the existence of a 'spiracular organ primordium' distinct from the established series of lateral line placodes ( Fig. 8 ), while a report in lungfishes (lobe-finned fishes) states that the spiracular organ primordium is unrelated to both lateral line and geniculate placodes [36] . Furthermore, the spiracular organ is exceptional both in its morphology and the distinctive central projections of its afferents: their primary projection area seems to overlap with ascending and descending octaval nuclei, and there are projections through and around these nuclei to lateral regions of the reticular formation that may be related to jaw movement or respiratory centres [9] . These unique features also suggest that the spiracular organ may be distinct from the lateral line and may function, like the ear, as a proprioceptor [31] . The putative developmental and evolutionary independence of the spiracular organ/PTO from the lateral line system is further supported by the fact that some anamniote groups (modern amphibians, teleosts) have independently lost the spiracular organ but retained the lateral line system, just as amniotes have retained the spiracular organ/PTO but lost the lateral line system. Developmental independence from the lateral line system combined with a proprioceptor function that is independent of water or air flow through the spiracle would have enabled its retention in the amniote ancestor, even as the lateral line system was lost. 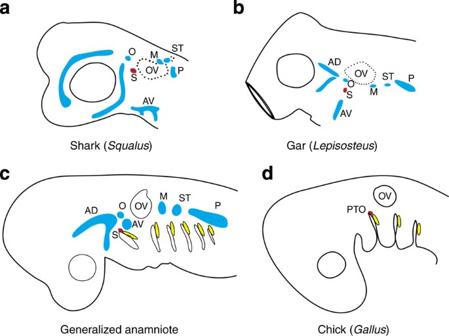Figure 8: Overview of vertebrate placodes derived from the 'posterior placodal area'. (a) Schematic summarizing data from a cartilaginous fish, the sharkSqualus acanthias33, redrawn from ref.48, suggesting the presence of a spiracular organ primordium (red) that is separate from the established series of six lateral line placodes (blue). (b) Schematic summarizing data from a non-teleost ray-finned fish, the longnose gar,Lepisosteus osseus34, redrawn from ref.48, also showing a separate spiracular organ primordium. Similar results were also reported for the shortnose gar,L. platystomus35. (c) Schematic (modified from ref.32) of a hypothetical generalized anamniote embryo, showing the proposed relationship between the otic vesicle (OV), lateral line placodes (blue), spiracular organ primordium (red) and epibranchial placodes (yellow). (d) Schematic of a pharyngula stage chicken embryo highlighting the position of the epibranchial (yellow) and PTO (red) placodes. AD, anterodorsal lateral line placode; AV, anteroventral lateral line placode; M, middle lateral line placode; O, otic lateral line placode; OV, otic vesicle; P, posterior lateral line placode; S, spiracular organ placode; ST, supratemporal lateral line placode. Figure 8: Overview of vertebrate placodes derived from the 'posterior placodal area'. ( a ) Schematic summarizing data from a cartilaginous fish, the shark Squalus acanthias [33] , redrawn from ref. 48 , suggesting the presence of a spiracular organ primordium (red) that is separate from the established series of six lateral line placodes (blue). ( b ) Schematic summarizing data from a non-teleost ray-finned fish, the longnose gar, Lepisosteus osseus [34] , redrawn from ref. 48 , also showing a separate spiracular organ primordium. Similar results were also reported for the shortnose gar, L. platystomus [35] . ( c ) Schematic (modified from ref. 32 ) of a hypothetical generalized anamniote embryo, showing the proposed relationship between the otic vesicle (OV), lateral line placodes (blue), spiracular organ primordium (red) and epibranchial placodes (yellow). ( d ) Schematic of a pharyngula stage chicken embryo highlighting the position of the epibranchial (yellow) and PTO (red) placodes. AD, anterodorsal lateral line placode; AV, anteroventral lateral line placode; M, middle lateral line placode; O, otic lateral line placode; OV, otic vesicle; P, posterior lateral line placode; S, spiracular organ placode; ST, supratemporal lateral line placode. Full size image Overall, we conclude that the amniote PTO is indeed homologous to the anamniote spiracular organ, originating (together with its afferent neurons) from a previously undiscovered placode lying dorsal to the geniculate placode. We suggest that, rather than the PTO being a lateral line remnant in amniotes, the spiracular organ/PTO and its cognate placode could represent an ancient developmental and evolutionary module, independent of both epibranchial and lateral line placodes. Embryos All studies were in full compliance with guidelines for the use of embryonic material at the RIKEN Center for Developmental Biology, University of Cambridge and University of Iowa, where this work took place. Fertilized chicken and quail eggs were obtained from commercial sources and incubated in a humidified incubator at 38 °C until the desired stage. Staging was performed using the normal staging tables published in ref. 16 , or by counting somites. Shark ( S. canicula ) embryos were provided by David Sims at the Marine Biological Association, Plymouth, UK, or by the University of Glasgow Biological Station, Millport, Isle of Cumbrae, UK; they were kept in oxygenated seawater at 15 °C and staged using the normal staging tables published in ref. 37 . Quail-chick grafting Quail donor embryos were explanted and pinned out in Ringer's solution and ectodermal tissues dissected using pulled glass needles. After windowing the eggshell, chicken host embryos were visualized in ovo by injecting Indian ink (diluted 1:10 in Ringer's solution) into the sub-blastodermal cavity. A small tear was made in the vitelline membrane, and the appropriate ectodermal region excised and replaced with donor quail tissue. Eggs were sealed with tape and returned to the incubator until the required stage. Surviving embryos were fixed in modified Carnoy's solution (six volumes ethanol: three volumes 37% formaldehyde: one volume glacial acetic acid) and processed for cryosectioning. Tissue culture Tissue chunks (ectoderm, mesoderm and endoderm) from the otocyst, peri-geniculate placode region (pre-otic, first pharyngeal cleft region), or petrosal placode region (post-otic, second pharyngeal cleft region), of stage 15–16 (24–28 somite stage; 50–56 h) chicken embryos ( Fig. 7h ) were excised using pulled glass needles in Ringer's solution. Explants were transferred to uncoated plastic Petri dishes flooded with DMEM/F12 (GIBCO) medium containing N2 and B27 supplements (GIBCO). Human BMP4 or BMP7 recombinant protein (R&D Systems) was added to a final concentration of 4 ng ml −1 . These 'floating' cultures were incubated for 5–7 days at 37 °C, then fixed overnight in 4% paraformaldehyde, washed in PBS with 0.05% Tween-20 and embedded for cryosectioning. Sectioning For cryosectioning, fixed specimens were rehydrated, then cryo-preserved by immersion in a series of graded (10, 20, 30%) sucrose solutions in PBS. Samples were frozen in liquid nitrogen after orientation in OCT (Sigma) and stored at −80 °C. Cryosections were cut at 10–12 μm and allowed to dry at room temperature for 1 h. Before immunostaining, thawed cryosections were immersed in PBT (PBS, 0.25% Tween-20) to remove excess OCT. For paraffin wax sectioning, embryos were dehydrated in three changes of 100% ethanol, transferred to Histosol (National Diagnostics) or Lemosol (Wako) for three 30-min washes, then infiltrated with paraffin wax (Raymond Lamb: three 1-h changes at 60°C). Samples were oriented in plastic moulds and sectioned at 10 μm onto Superfrost Plus slides (Fisher Scientific) using a rotary microtome. Haematoxylin and eosin (H&E) staining Slides were immersed in Mayer's haematoxylin (Muto Pure Chemicals) for 10 min then washed for 5 min in running tap water. Slides were briefly dipped in acid alcohol solution (5% acetic acid, 95% ethanol) to destain haematoxylin to a suitable intensity. After immersion in 0.5% eosin Y solution (Sigma) for 2 min, they were returned to flowing tap water for ~ 1 min, then placed in 95% ethanol for 1 min, then 100% ethanol for 3 min, before finally being transferred to Lemosol (Wako) and mounted using DPX (Merck). Immunohistochemistry on sections Slides were blocked using 10% goat serum in PBT for 1 h at room temperature. Primary antibodies were applied overnight at 4 °C in PBT as follows: 1 in 500 anti-Brn3a [38] , [39] (mouse IgG1, Millipore); 1 in 200 anti-Brn3a [40] (guinea-pig, kind gift of Eric Turner, Seattle Children's Research Institute, USA); 1 in 2,000 anti-HCA/Ptprq (rabbit; kind gift of Guy Richardson, University of Sussex, UK); 1 in 500 anti-Islet1 (mouse IgG2b; clone 39.4D5 from Developmental Studies Hybridoma Bank, DSHB); 1 in 500 anti-laminin (rabbit; Sigma); 1 in 2,000 anti-myosin-VI (rabbit; Abcam); 1 in 1,000 anti-myosin-VII (rabbit, kind gift of Christine Petit, Institut Pasteur, France); 1 in 500 anti-Pax2 (rabbit; Zymed/Invitrogen); 1 in 400 anti-PROX1 (rabbit; Covance); 1 in 500 anti-Sox2 (rabbit; Chemicon); 1 in 500 anti-Sox2 (mouse IgG1; Abcam); 1 in 500 anti-Sox3 (rabbit, kind gift of Sara Wilson, Umeå University, Sweden); 1 in 500 anti-neuronal beta-III tubulin (Tuj1, mouse IgG2a; Covance); 1 in 2 anti-quail cells (QCPN, mouse IgG1; DSHB); 1 in 2 anti-quail neurites (QN [41] , mouse IgG1; kind gift of Hideaki Tanaka, Kumamoto University, Japan). For double Brn3a/QCPN staining, 1 in 50 Alexa 568 -conjugated QCPN was used (kind gift of Marianne Bronner-Fraser, CalTech, USA). (The DSHB was developed under the auspices of the NICHD and is maintained by the University of Iowa, Department of Biological Sciences, Iowa City.) After three 20-min washes in PBT, appropriate fluorescent secondary antibodies (Invitrogen), diluted 1/1,000 in 10% goat serum in PBT, were applied for 2 h at room temperature. Finally, sections were washed in PBT, counterstained for 3 min with DAPI (Dojindo, Japan, 1 in 4,000 dilution) and mounted in Aqua Polymount (Polysciences) for viewing under epifluorescence. In situ hybridization on cryosections Embryonic heads were fixed in 4% paraformaldehyde overnight at 4 °C, rinsed extensively in PBS and embedded for cryosectioning at 15–20 μm as described above. In situ hybridization was performed as described previously for wax sections [42] , omitting the dewaxing and rehydration steps necessary for wax sections. Bmp7 was a gift from Marianne Bronner-Fraser (CalTech, USA). Bmp4 was a gift from Eldad Tzahor (Weizmann Institute of Science, Israel). Atonal1 (ChEST496o6) was obtained from the BBSRC ChickEST database ( http://www.chick.manchester.ac.uk/ ). SOHo1 was used as in ref. 43 . A 700-base pair fragment of chick Sox3 (NM_204195.1) including 300 base pairs of the 3′ untranslated region was cloned from cDNA and used to generate riboprobe. Whole mount in situ hybridization For detecting Sox2 , Pax2 , Sox3 and Delta1 transcripts, embryonic chick heads were fixed in 4% paraformaldehyde, bisected along the midline and neural tube tissue was removed. In situ hybridization was performed as described in ref. 43 . NeuroVue dye labelling Lipophilic dyes (NeuroVue Maroon, Red; available from Molecular Targeting Technologies, Inc.) were applied in solid form (to avoid spreading) into the ear, PTO or branches of the facial nerve of stage 27–31 (E5–7) embryos to label single or multiple afferents to the brain. In addition, dyes were inserted into ascending and descending inner ear and facial nerve projections to label afferents to the ear, the PTO and the facial nerve. Brains and skulls were dissected, mounted in glycerol and viewed with a Leica SP5 confocal microscope. Three-dimensional reconstruction Serial sections of H&E-stained stage 25 (E4.5) chick head were imaged and used as input for SPIERS (Serial Palaeontological Image Editing and Rendering System) software ( http://spiers-software.org/ ). How to cite this article: O'Neill, P. et al . The amniote paratympanic organ develops from a previously undiscovered sensory placode. Nat. Commun. 3:1041 doi: 10.1038/ncomms2036 (2012).